Optogenetic analysis of synaptic transmission in the central nervous system of the nematodeCaenorhabditis elegans A reliable method for recording evoked synaptic events in identified neurons in Caenorhabditis elegans would greatly accelerate our understanding of its nervous system at the molecular, cellular and network levels. Here we describe a method for recording synaptic currents and potentials from identified neurons in nearly intact worms. Dissection and exposure of postsynaptic neurons is facilitated by microfabricated agar substrates, and ChannelRhodopsin-2 is used to stimulate presynaptic neurons. We used the method to analyse functional connectivity between a polymodal nociceptor and a command neuron that initiates a stochastic escape behaviour. We find that escape probability mirrors the time course of synaptic current in the command neuron. Moreover, synaptic input increases smoothly as stimulus strength is increased, suggesting that the overall input–output function of the connection is graded. We propose a model in which the energetic cost of escape behaviours in C. elegans is tuned to the intensity of the threat. Any method for synaptic physiology between identified neurons should allow for selective stimulation of the presynaptic neuron, quantitative control of presynaptic activation and positive identification of the postsynaptic neuron. In many systems, these requirements can be met by making pairwise whole-cell patch-clamp recordings. Such pairwise recordings are challenging in any system, but in Caenorhabditis elegans the challenge is compounded by the fact that whole-cell patch-clamp recordings from individual neurons are comparatively short-lived. In genetically tractable organisms, however, the first two requirements can now be met using an optogenetic approach in which a photoactivatable ion channel is genetically targeted to the desired presynaptic neurons [1] , [2] , [3] , [4] . The third requirement can be met by targeting the expression of fluorescent proteins to the desired postsynaptic neurons [5] . To develop such a method in C. elegans , we focused on the connection between the neuron classes ASH and AVA. ASH is a left–right pair of glutamatergic, nociceptive sensory neurons [6] , [7] , [8] , [9] , [10] , [11] . Anatomical reconstructions imply that ASH makes monosynaptic and polysynaptic connections onto AVA, a left–right pair of premotor command interneurons that expresses at least two types of glutamate receptors [12] , [13] , [14] , [15] , [16] . Our selection of the ASH–AVA connection was based on three main considerations. First, there is ample physiological evidence that the connection is functional as mechanical and optical stimulation of ASH elicits inward synaptic currents and calcium transients in AVA, respectively [17] , [18] . Second, ASH makes monosynaptic connections onto AVA [16] . Third, the connection is behaviourally relevant, as ASH neurons respond to stimuli that elicit escape responses [8] , and AVA neurons are required for, and are active during, reverse locomotion [14] , [19] , an inherent component of escape behaviours in C. elegans . Here we present a method for recording quantitatively evoked synaptic currents and potentials at central synapses in C. elegans for the first time. ChannelRhodopsin-2 (ChR2) is used to photoactivate [2] presynaptic neurons and the whole-cell patch-clamp configuration is used to record from postsynaptic neurons. To demonstrate the utility of the new methodology, we analysed synaptic correlates of AVA-mediated escape responses. We found that the time course of excitatory synaptic currents in AVA closely matched the time course of the probability of escape behaviour. Evoked currents were surprisingly complex, exhibiting three distinct components. The two main components increased smoothly as stimulus strength was increased, suggesting that the overall input–output function of AVA-mediated escape responses is graded. This result is consistent with a model in which the energetic cost of escape behaviours in C. elegans is tuned to the intensity of the threat. Optogenetics and neuronal identification To activate presynaptic neurons, we created a transgenic strain (XL165) in which ChR2, tagged with yellow fluorescent protein (YFP), is expressed under the control of the sra-6 promoter. This promoter was chosen because it has the greatest known specificity for ASH neurons. As expected from published sra-6 expression patterns [11] , we observed strong ChR2 expression in ASH and weak ChR2 expression in ASI, a left–right pair of chemosensory neurons required for diet-induced longevity, dauer formation, regulation of reverse locomotion, and chemotaxis [20] , [21] , [22] ; we refer to ASH and ASI collectively as ' sra-6 -expressing neurons.' Although photostimulation is likely to activate both pairs of neurons, the synaptic current attributable to ASI is likely to be small relative to the current attributable to ASH because of the difference in expression levels. The effectiveness of photostimulation was assessed in whole-cell patch-clamp recordings from ASH ( Fig. 1a,b ), which revealed an inward current with the transient and sustained components that are characteristic of this probe [3] . The amplitude and time course of the photocurrents were functions of stimulus irradiance, consistent with previous results in other systems [4] , as well as muscles and other neurons in C. elegans [2] , [23] . Photostimulation failed to elicit currents in worms grown in the absence of all- trans retinal, the essential cofactor [2] for ChR2, indicating that native light sensitivity in C. elegans [24] , [25] did not contribute to the currents recorded in ASH neurons at the irradiances used here. 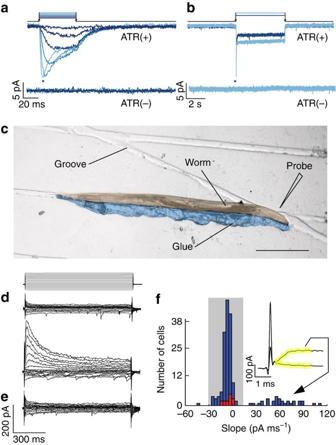Figure 1: Photostimulation of ASH neurons and electrophysiological identification of AVA neurons. (a) Membrane current evoked by photostimulation of ASH neurons with 50 ms long stimuli; asterisks denote the transient component of the current. The stimulus irradiance varied from 0.07 to 12.5 mW mm−2in steps of 1.04 log units. (b) Membrane current in ASH neurons in response to 5-s-long pulses of light at 0.75 and 12.5 mW mm−2. Upper and lower current traces are from animals supplied (ATR+) or not supplied (ATR−) with all-transretinal, respectively. Holding potential was −55 mV. (c) A glued worm positioned for dissection on a micropatterned agarose substrate. The worm and glue have been pseudocoloured to enhance contrast. Scale bar=200 μm. (d) Representatives of the two types of current families obtained when recording from unidentified command neurons presumed to be either AVA or AVE as identified by cell body position and expression of tdTomato driven by thenmr-1promoter. Voltage steps ranged from −80 to +40 mV in steps of 10 mV from a holding potential of −55 mV as shown above. (e) A current family from an AVA neuron positively identified by combinatorial expression of dsRed and GFP driven by theglr-1andrig-3promoters, respectively. The voltage protocol was the same as ind. (f) Histogram of the slope of the initial current in response the +40 mV voltage step in a population of 182 unidentified neurons that were either AVA or AVE (blue bars) and 10 neurons positively identified as AVA by combinatorial expression. Slope was computed over the 2 ms window (yellow) following termination of the capacitative transient; the inset shows typical traces during this window for the two types of current families shown ind. Shading indicates the subpopulation of neurons identifiedpost hocas AVA. Figure 1: Photostimulation of ASH neurons and electrophysiological identification of AVA neurons. ( a ) Membrane current evoked by photostimulation of ASH neurons with 50 ms long stimuli; asterisks denote the transient component of the current. The stimulus irradiance varied from 0.07 to 12.5 mW mm −2 in steps of 1.04 log units. ( b ) Membrane current in ASH neurons in response to 5-s-long pulses of light at 0.75 and 12.5 mW mm −2 . Upper and lower current traces are from animals supplied (ATR+) or not supplied (ATR−) with all- trans retinal, respectively. Holding potential was −55 mV. ( c ) A glued worm positioned for dissection on a micropatterned agarose substrate. The worm and glue have been pseudocoloured to enhance contrast. Scale bar=200 μm. ( d ) Representatives of the two types of current families obtained when recording from unidentified command neurons presumed to be either AVA or AVE as identified by cell body position and expression of tdTomato driven by the nmr-1 promoter. Voltage steps ranged from −80 to +40 mV in steps of 10 mV from a holding potential of −55 mV as shown above. ( e ) A current family from an AVA neuron positively identified by combinatorial expression of dsRed and GFP driven by the glr-1 and rig-3 promoters, respectively. The voltage protocol was the same as in d . ( f ) Histogram of the slope of the initial current in response the +40 mV voltage step in a population of 182 unidentified neurons that were either AVA or AVE (blue bars) and 10 neurons positively identified as AVA by combinatorial expression. Slope was computed over the 2 ms window (yellow) following termination of the capacitative transient; the inset shows typical traces during this window for the two types of current families shown in d . Shading indicates the subpopulation of neurons identified post hoc as AVA. Full size image The two standard methods for exposing C. elegans neurons for patch-clamp recording [12] , [26] , [27] involve large incisions in the cuticle and a sudden release of internal pressure, either of which might disrupt synaptic connections. We found that the preparation's physical integrity could be preserved to a greater degree by a new dissection procedure in which a tiny slit, less than 10 μm in length, is made immediately adjacent to the target neuron (AVA). In most instances, only a single neuron emerges from the slit. To facilitate this procedure, we manipulated worms before dissection into grooves formed in an agarose surface using a microfabricated mould ( Fig. 1c ) and glued them in place such that the worm's cuticle was convex at the point nearest to the target neuron. Postsynaptic neurons were identified for patch-clamp recording by transgenic expression of a red fluorescent protein (RFP), which is visualized by green light. Although we also tried green fluorescent protein (GFP) for this purpose, we found that the likelihood of observing evoked synaptic currents was much lower than when RFP was used, presumably because the blue light used to visualize GFP depresses synaptic transmission by sustained excitation of ChR2. Postsynaptic neurons were identified by expression of the RFP known as tdTomato [28] under the control of the nmr-1 promoter, which labels the command neuron AVA, its nearest neighbour AVE, and four other interneurons that are further away [12] . Although AVA and AVE can be distinguished, in principle, by the relative positions of their somata, it was not always possible to discern which neuron emerged from the slit. However, inspection of the amplitude and time course of the current families measured in voltage clamp, when either of the two neurons may have been exposed, revealed two qualitatively distinct physiological types: one having small currents that activated almost instantaneously and decayed quickly, and the other having large currents that activated and decayed more slowly ( Fig. 1d ). We also noted that the whole-cell capacitance in recordings of the first type was systematically larger than the whole-cell capacitance in the second type (0.77±0.02 versus 0.53±0.02 pF; P <0.001). This result suggested that the first type corresponds to AVA neurons, whose only neurite is twice as long as that of AVE [16] . We confirmed this correspondence by recording from a transgenic strain in which AVA could be identified positively as the only neuron that expressed both a red and a green fluorescent protein marker ( Fig. 1e,f ). Henceforth, we identified AVA by its unambiguous physiological characteristics alone, using the initial slope of the membrane current as shown in Figure 1f . Escape responses elicited by photostimulation Before trying to record synaptic currents in AVA neurons in the strain XL165, we tested whether AVA neurons are likely to exhibit synaptic responses in this strain by attempting to elicit escape responses via photostimulation. These experiments were done using the so-called glued-worm preparation [29] , [30] , in which the worm is glued by the head to an agarose-coated coverslip and bouts of reverse locomotion ('reversals') are scored manually by noting the direction of propagation of undulatory waves along the worm's body. To ensure that photostimulation was the same as in the electrophysiological experiments recounted below, we performed the behavioural assays in our patch-clamp setup, using its light source and microscope objective for photostimulation. As expected, reversal bouts occurred stochastically [31] , [32] before, during and after photostimulation ( Fig. 2a ). However, plotting the change in the probability of reverse locomotion versus time ( Fig. 2b ) revealed clear increases in probability for two of the three stimulus strengths used; the third stimulus was apparently too weak to elicit detectable behaviour. Because AVA makes a major contribution to reversals [14] , these results provided some assurance that synaptic responses would be seen in patch-clamp recordings from AVA. 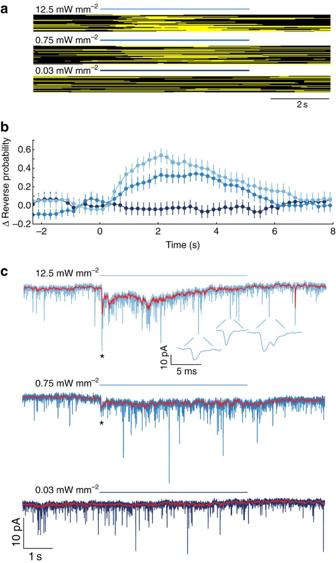Figure 2: Time course of reversal behaviour and the synaptic current in AVA evoked by photostimulation ofsra-6-expressing neurons. (a) Raster plots showing the behavioural state of semi-restrained worms in response to photostimulation at three different irradiances. Black and yellow pixels indicate forward and reverse swimming, respectively. Blue bars show the time of the photostimulus at the indicated irradiance. (b) The stimulus evoked change in the probability of reverse swimming for the data shown ina. Error bars are s.e.m. (n>42 for each stimulus condition). (c) Typical synaptic current in AVA evoked by photostimulation ofsra-6-expressing neurons at the three irradiances shown ina. Holding potential was −55 mV. Three phenomenologically distinct components of the response are visible: the onset transient (asterisk), the sustained current (red trace showing median-filtered current), and the increase in the unitary event frequency (insets). Data ina–care plotted on the same time axis to facilitate comparison of the time course of behaviour and synaptic current. Figure 2: Time course of reversal behaviour and the synaptic current in AVA evoked by photostimulation of sra-6 -expressing neurons. ( a ) Raster plots showing the behavioural state of semi-restrained worms in response to photostimulation at three different irradiances. Black and yellow pixels indicate forward and reverse swimming, respectively. Blue bars show the time of the photostimulus at the indicated irradiance. ( b ) The stimulus evoked change in the probability of reverse swimming for the data shown in a . Error bars are s.e.m. ( n >42 for each stimulus condition). ( c ) Typical synaptic current in AVA evoked by photostimulation of sra-6 -expressing neurons at the three irradiances shown in a . Holding potential was −55 mV. Three phenomenologically distinct components of the response are visible: the onset transient (asterisk), the sustained current (red trace showing median-filtered current), and the increase in the unitary event frequency (insets). Data in a – c are plotted on the same time axis to facilitate comparison of the time course of behaviour and synaptic current. Full size image Synaptic currents in AVA neurons To investigate the relationship between synaptic input to AVA and the time course of reversal responses, we recorded synaptic currents in AVA in response to light pulses that matched the duration and irradiance of the light pulses used in the behavioural experiments of Figure 2a,b . Synaptic currents elicited by photostimulation were inward ( Fig. 2c ), consistent with the fact that ASH is a glutamatergic neuron, and AVA is known to express ionotropic glutamate receptors and to exhibit an inward current in response to direct application of glutamate in dissected preparations [12] , [15] , [17] . It should also be noted that laser ablations of ASI indicate that it normally acts to suppress reversal behaviour [22] , suggesting that the inward currents we observed in AVA are attributable solely to ASH. This fact, together with the above-mentioned contrast between ChR2 expression levels in ASH and ASI, suggests that the effect of ASI activation is at most a modest reduction in the amplitude of this inward current. Thus, photostimulation of sra-6 -expressing neurons appears to be a reasonable approximation to photostimulation of ASH alone. Synaptic currents in AVA were remarkably well correlated with reversal behaviour (measured in different animals) in three important respects. First, currents were observed in response to the two stimuli that were behaviourally sufficient, whereas currents were absent in response to the only stimulus that was behaviourally insufficient. Second, the stimulus that elicited the strongest behavioural response also elicited the strongest synaptic response. Third, the overall duration of the currents matched the duration of the behavioural responses. We conclude that synaptic current in AVA is well correlated with reversal probability. Further inspection of AVA synaptic currents revealed three phenomenologically distinct components. The first component ('onset transient,' Fig. 2c , asterisks) was a short-latency current that decayed rapidly. Synaptic latency, measured relative to the onset of the light pulse (see Methods ), was a decreasing function of stimulus irradiance ( Supplementary Fig. S1 ). 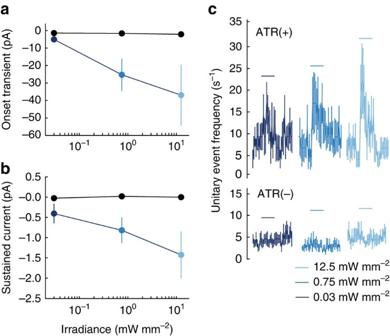Figure 3: Quantitative summary of the three components of the synaptic current in AVA evoked by photostimulation ofsra-6-expressing neurons. Currents were quantified and subjected to an analysis of variance to test for a linear relationship with irradiance. (a) Peak onset transient synaptic current versus irradiance in animals supplied with all-transretinal (ATR(+), blue dots,n=9) and retinal-free controls (ATR(−), black dots,n=4). The magnitude of the onset transient from ATR(+) animals increased significantly with stimulus irradiance (P=0.029). (b) Average sustained synaptic current versus irradiance. Current was averaged over the interval 0≤t≤2.1 s. Symbols as ina. The magnitude of sustained currents from ATR(+) animals increased significantly with stimulus irradiance (P=0.044). (c) Average time course of the frequency of unitary synaptic events in response to photostimulation at three different irradiances (horizontal blue bars). The frequency of unitary synaptic events evoked by photostimulaion increased with stimulus irradiance in ATR(+) animals, but this effect did not reach significance (ANOVA,P=0.246). Upper and lower traces show data from animals supplied or not supplied with all-transretinal, respectively. ATR(+)n=9, ATR(−)n=4. Error bars (a–c) are s.e.m. Statistics (a–c): within-subjects ANOVA test for a linear trend. The peak amplitude of the onset transient was an increasing function of stimulus irradiance as shown by the current–irradiance plot in Figure 3a . The second component ('sustained current,' Fig. 2c , red trace) was a long-lived current identified in the figure by median filtering of the membrane current. To quantify this component, we computed its average during the time period corresponding to the rising phase of the behavioural responses shown in Figure 2b (0≤ t ≤2.1 s); it too was found to be an increasing function of irradiance ( Fig. 3b ). The third component ('unitary event frequency', Fig. 2c , insets) was a transient increase in the frequency of small, unitary synaptic currents. The effect on this component of increasing stimulus irradiance was not statistically significant ( Fig. 3c ). We conclude that the onset and sustained components of the synaptic current observed in response to photostimulation are graded functions of stimulus strength. Figure 3: Quantitative summary of the three components of the synaptic current in AVA evoked by photostimulation of sra-6 -expressing neurons. Currents were quantified and subjected to an analysis of variance to test for a linear relationship with irradiance. ( a ) Peak onset transient synaptic current versus irradiance in animals supplied with all- trans retinal (ATR(+), blue dots, n =9) and retinal-free controls (ATR(−), black dots, n =4). The magnitude of the onset transient from ATR(+) animals increased significantly with stimulus irradiance ( P =0.029). ( b ) Average sustained synaptic current versus irradiance. Current was averaged over the interval 0≤ t ≤2.1 s. Symbols as in a . The magnitude of sustained currents from ATR(+) animals increased significantly with stimulus irradiance ( P =0.044). ( c ) Average time course of the frequency of unitary synaptic events in response to photostimulation at three different irradiances (horizontal blue bars). The frequency of unitary synaptic events evoked by photostimulaion increased with stimulus irradiance in ATR(+) animals, but this effect did not reach significance (ANOVA, P =0.246). Upper and lower traces show data from animals supplied or not supplied with all- trans retinal, respectively. ATR(+) n =9, ATR(−) n =4. Error bars ( a – c ) are s.e.m. Statistics ( a – c ): within-subjects ANOVA test for a linear trend. Full size image Evidence for graded synaptic connectivity between ASH and AVA As we understand the term, a 'graded synaptic connection' is one in which action potentials are required neither for transmitter release nor for postsynaptic signalling, and in which incremental changes in membrane potential in the soma of the presynaptic neuron cause incremental changes in membrane potential in the soma of the postsynaptic neuron [33] . This term can be applied to monosynaptic connections and to so-called functional connections, which are defined in terms of the net effect of multiple synaptic pathways, including parallel pathways that may also be polysynaptic. The signature of a graded synaptic connection is a smoothly rising input–output function, defined by the curve obtained when postsynaptic membrane potential is plotted against presynaptic membrane potential. Conversely, the signature of a non-graded synaptic connection is an input–output function that exhibits a step-like discontinuity, indicating a distinct threshold for synaptic transmission. To delineate the approximate input–output function of the connection between ASH and AVA, we recorded voltage responses in these neurons, when ASH was stimulated by an increasing series of brief (50 ms) light pulses. We found that the amplitudes of responses of ASH and AVA to photostimulation were increasing functions of stimulus irradiance and lacked any discontinuities that might suggest non-graded synaptic transmission. This relationship held for presynaptic depolarizations in ASH ( Fig. 4a,b ), postsynaptic currents in AVA ( Fig. 4c,d ) and postsynaptic potentials in AVA ( Fig. 4e,f ). Discontinuities were also absent when, combining data from both experiments, we plotted postsynaptic membrane potential against presynaptic membrane potential ( Fig. 4g ), in accordance with the definition of a graded synaptic connection. Together, these data are consistent with a graded functional synaptic connection between ASH and AVA. This finding agrees with previous reports of graded synaptic transmission between neurons in the nematode Ascaris suum and at the neuromuscular junction in Ascaris suum and C. elegans [23] , [34] , [35] . 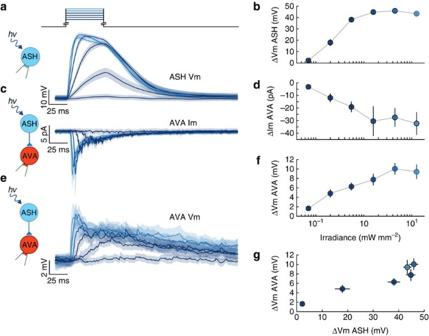Figure 4: Evidence for graded synaptic transmission betweensra-6-expressing neurons and the command neuron AVA. (a) Average membrane potential of ASH neurons in response to the photostimulation protocol shown at the top. Colour indicates stimulus irradiance which varied from 0.07 to 12.5 mW mm−2in steps of 1.04 log units. (b) Peak depolarization evoked in ASH versus irradiance (n=14 ina,b). (c) Average membrane current in AVA neurons (photostimulation as ina). (d) Peak synaptic current evoked in AVA versus irradiance (n=9 inc,d). (e) Average membrane potential in AVA neurons (photostimulation as ina). (f) Peak synaptic potential versus stimulus irradiance (n=18 ine,f). Data were recorded from the indicated neuron but in different animals. (g) Postsynaptic membrane potential infplotted against presynaptic membrane potential ind. s.e.m. is indicated by gray bands ina,c,d, and error bars inb,d,f,g. Figure 4: Evidence for graded synaptic transmission between sra-6 -expressing neurons and the command neuron AVA. ( a ) Average membrane potential of ASH neurons in response to the photostimulation protocol shown at the top. Colour indicates stimulus irradiance which varied from 0.07 to 12.5 mW mm −2 in steps of 1.04 log units. ( b ) Peak depolarization evoked in ASH versus irradiance ( n =14 in a , b ). ( c ) Average membrane current in AVA neurons (photostimulation as in a ). ( d ) Peak synaptic current evoked in AVA versus irradiance ( n =9 in c , d ). ( e ) Average membrane potential in AVA neurons (photostimulation as in a ). ( f ) Peak synaptic potential versus stimulus irradiance ( n =18 in e , f ). Data were recorded from the indicated neuron but in different animals. ( g ) Postsynaptic membrane potential in f plotted against presynaptic membrane potential in d . s.e.m. is indicated by gray bands in a , c , d , and error bars in b , d , f , g . Full size image The design of the experiment in Figure 4 also allowed us to compare the time course of synaptic currents and synaptic potentials in AVA neurons, albeit in different animals. It is interesting to note that average synaptic potentials outlasted average synaptic current evoked by the same photostimulus ( Fig. 4c versus e). Temporal filtering by passive membrane properties of AVA neurons was not sufficient to account for this discrepancy, as the average predicted membrane time constant of AVA neurons was 0.85±0.03 ms (see Methods ). This result suggests that synaptic potentials in AVA may involve one or more types of sustained postsynaptic mechanisms. Possibilities include cellular-level mechanisms such as current through N -methyl D -aspartate (NMDA) receptors expressed in AVA neurons [12] or network-level mechanisms such as positive feedback via recurrent excitatory synaptic connections [16] . Further experiments will be required to distinguish between these possibilities. Distinguishing between chemical and electrical transmission Gap junctions, the anatomical correlates of electrical synapses, are commonly encountered in the reconstructions of C. elegans central nervous system [16] . To test whether the synaptic current between sra-6 -expressing neurons and AVA contains an electrical component, we attempted to record synaptic currents in mutant worms in which classical chemical synaptic transmission is known to have been essentially eliminated by a loss-of-function mutation in the gene unc-13 . This gene encodes the nematode form of MUNC-13, which is required for the priming and release of clear-core vesicles characteristic of synapses that utilize glutamate and other classical neurotransmitters [36] , [37] . We found that all three components of the synaptic current, evoked by photo-simulation of sra-6 -expressing neurons, were absent in unc-13 ( e51 ) mutants ( Fig. 5 ), leading us to conclude that pathways consisting of purely electrical synapses do not make a detectable contribution to evoked synaptic currents in AVA. We also found that the unc-13 ( e51 ) mutation eliminated the spontaneous events seen in the baseline periods before photostimulation ( Fig. 5a,b,d ), indicating that these events too are synaptic in origin. Together, these findings are consistent with the fact that the C. elegans neuronal connectivity database shows that there are only a few all-electrical synaptic pathways from sra-6 -expressing neurons to AVA and all of them are highly indirect (fifth order or higher) [16] . The absence of evoked synaptic currents in unc-13 mutants does not, of course, rule out a contribution from polysynaptic pathways that contain both chemical and electrical synapses. 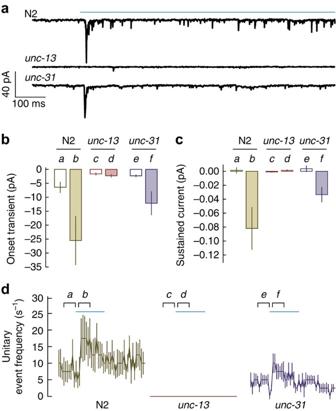Figure 5: Synaptic currents evoked by photostimulation ofsra-6-expressing neurons in two synaptic transmission mutants. (a) Typical currents in wild-type (N2) animals and animals with mutations in synaptic transmission mediated by clear-core vesicles (unc-13(e51)) or dense-core vesicles (unc-31(e928)). The photostimulus is shown by the blue bar above the top trace. (b) Summary of effects on the onset transient. Theunc-13mutation eliminated the onset transient (bversusd,P=0.002) whereas theunc-31mutation did not have a significant effect (bversusf,P=0.2978). (c) Summary of effects on the sustained current. Theunc-13mutation eliminated the sustained current (bversusd,P=0.00025) whereas theunc-31mutation did not have a significant effect (bversusf,P=0.652). (d) Summary of effects on frequency of unitary events relative to stimulus onset in wild type. Theunc-13mutation essentially eliminated the increase in unitary event frequency (bversusd,P=0.0002) whereas theunc-31 mutation did not have a significant effect (bversusf,P=0.037). Statistics (b–d): Bonferroni-adjusted Mann–WhitneyU-test. The joint level of significance (α) in the Bonferroni adjustment was 0.017 inb, and 0.025 inc,d. Sample sizes were: wild type,n=9;unc-13,n=10; andunc-31,n=10. Error bars are s.e.m. Figure 5: Synaptic currents evoked by photostimulation of sra-6 -expressing neurons in two synaptic transmission mutants. ( a ) Typical currents in wild-type (N2) animals and animals with mutations in synaptic transmission mediated by clear-core vesicles ( unc-13 ( e51 )) or dense-core vesicles ( unc-31 ( e928 )). The photostimulus is shown by the blue bar above the top trace. ( b ) Summary of effects on the onset transient. The unc-13 mutation eliminated the onset transient ( b versus d , P =0.002) whereas the unc-31 mutation did not have a significant effect ( b versus f , P =0.2978). ( c ) Summary of effects on the sustained current. The unc-13 mutation eliminated the sustained current ( b versus d , P =0.00025) whereas the unc-31 mutation did not have a significant effect ( b versus f , P =0.652). ( d ) Summary of effects on frequency of unitary events relative to stimulus onset in wild type. The unc-13 mutation essentially eliminated the increase in unitary event frequency ( b versus d , P =0.0002) whereas the unc -31 mutation did not have a significant effect ( b versus f , P =0.037). Statistics ( b – d ): Bonferroni-adjusted Mann–Whitney U -test. The joint level of significance (α) in the Bonferroni adjustment was 0.017 in b , and 0.025 in c , d . Sample sizes were: wild type, n =9; unc-13 , n =10; and unc-31 , n =10. Error bars are s.e.m. Full size image In addition to clear-core synaptic vesicles, C. elegans neurons also contain so-called dense core vesicles, which release catecholamines and neuropeptides [38] . Although ASH is not known to express synthetic enzymes for catecholamines [39] , it does express genes for at least four neuropeptides, and neuropeptide gene expression is also seen in neurons that are members of the polysynaptic pathways between ASH and AVA. To test whether a component of the synaptic current in AVA might involve the release of dense-core vesicles, we recorded synaptic currents in mutants in which this release mechanism has been impaired by a deletion ( e928 ) in the gene unc-31 , which is required for all dense-core vesicle release in C. elegans [40] , [41] . Although we observed a trend towards reduction of synaptic currents across all three components ( Fig. 5 ), the effect failed to reach significance for any individual component. We conclude that there might be a modest requirement for UNC-31 in synaptic signalling between ASH and AVA, suggesting a possible role for peptides and catecholamines as neurotransmitters or neuromodulators. A similarly mild effect has been observed in null mutants of the analogous gene in Drosophila [42] . Evidence for glutamate transmission Candidate glutamatergic synapses in C. elegans can be identified using genetic evidence for presynaptic expression of the glutamate vesicular transporter gene eat-4 (ref. 6 ), together with postsynaptic expression of NMDA or non-NMDA glutamate receptor subunits [15] , [43] . One such candidate is the monosynaptic connection from ASH to AVA. The observation that AVA neurons exhibit inward currents in response to exogenously applied glutamate [15] , [17] supports this view. However, glutamatergic synapses are likely to have a central role in polysynaptic connections as well. Indeed, by combining the C. elegans neuronal wiring diagram with published expression patterns of eat-4 and various glutamate receptor subunits [6] , [44] , we found that 62 of the 72 polysynaptic pathways (up to fourth order) between ASH and AVA contain at least one connection that is a candidate glutamatergic synapse. As a direct test of whether glutamatergic transmission is required for the connectivity between ASH and AVA, we first measured the peak current–voltage relationship of the synaptic currents elicited in AVA by photostimulation of sra-6 -expressing neurons ( Fig. 6a,b ). We found that synaptic currents reversed near 0 mV, the value obtained in recordings from AVA neurons in dissected preparations in response to exogenous glutamate [17] . We next recorded synaptic currents in the combined presence of the glutamate antagonists CNQX (6-cyano-7-nitroquinoxaline-2,3-dione) and MK-801. We found that glutamate antagonists reduced the amplitude of all three components of the AVA synaptic current ( Fig. 6c–f ). Together, these findings lead us to conclude that the overall connectivity between ASH and AVA is at least partly glutamatergic. The persistence of synaptic currents in the presence of glutamate antagonists may reflect a glutamate-independent component of the synaptic current or incomplete access of the antagonists to the central nervous system. The latter might be expected because the hole formed in the cuticle during dissection is small and likely to be partially occluded by surrounding soft tissue. 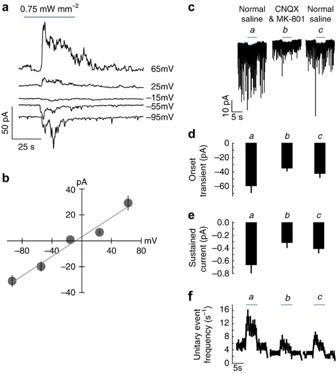Figure 6: Evidence for glutamatergic synaptic transmission betweensra-6-expressing neurons and AVA. (a) Reversal of synaptic currents in AVA by clamping the neuron at holding potentials from −95 to +65 mV. (b) Peak synaptic current versus holding potential in 10 AVA neurons. A linear fit indicates a reversal potential of −7.0±3.2 mV. (c) Typical spontaneous and evoked synaptic currents recorded from AVA in normal saline, during the bath application of glutamate blockers CNQX (200 μM) and MK-801 (50 μM), and following washout with normal saline. The photo stimulus is indicated by the blue bar. (d) Glutamate blockers reduced the average onset transient during the stimulus (pooleda,cversusb,P=0.0009;aversusc,P=0.622). (e) Glutamate blockers reduced the average sustained current during the stimulus (pooleda,cversusb,P=0.0007;aversusc,P=0.575). (f) Glutamate blockers reduced the average unitary event frequency during the stimulus (pooleda,cversusb,P=0.003;aversusc,P=0.375). Statistics (d–f): within-subjects analysis of variance (n=10) with orthogonal planned comparisons. The joint level of significance (α) was 0.025 throughout. Error bars are s.e.m. CNQX, 6-cyano-7-nitroquinoxaline-2,3-dione. Figure 6: Evidence for glutamatergic synaptic transmission between sra-6 -expressing neurons and AVA. ( a ) Reversal of synaptic currents in AVA by clamping the neuron at holding potentials from −95 to +65 mV. ( b ) Peak synaptic current versus holding potential in 10 AVA neurons. A linear fit indicates a reversal potential of −7.0±3.2 mV. ( c ) Typical spontaneous and evoked synaptic currents recorded from AVA in normal saline, during the bath application of glutamate blockers CNQX (200 μM) and MK-801 (50 μM), and following washout with normal saline. The photo stimulus is indicated by the blue bar. ( d ) Glutamate blockers reduced the average onset transient during the stimulus (pooled a , c versus b , P =0.0009; a versus c , P =0.622). ( e ) Glutamate blockers reduced the average sustained current during the stimulus (pooled a , c versus b , P =0.0007; a versus c , P =0.575). ( f ) Glutamate blockers reduced the average unitary event frequency during the stimulus (pooled a , c versus b , P =0.003; a versus c , P =0.375). Statistics ( d – f ): within-subjects analysis of variance ( n =10) with orthogonal planned comparisons. The joint level of significance (α) was 0.025 throughout. Error bars are s.e.m. CNQX, 6-cyano-7-nitroquinoxaline-2,3-dione. Full size image Although the present combination of photostimulation and patch-clamp electrophysiology ('photo-electrophysiology') has been used effectively in studies of synaptic transmission at the C. elegans neuromuscular junction [1] , [23] , it has not been applied to synapses of the central nervous system in C. elegans until now. A key feature of the new method is a minimally invasive dissection procedure designed to increase the likelihood that synaptic connections remain intact after the cell body of the postsynaptic neuron is exposed for recording. This procedure was facilitated by gluing the animals in close-fitting grooves formed by a microfabricated mould. The main limitation of photo-electrophysiology in C. elegans is the current scarcity of pairs of promoters that are entirely specific for the presynaptic and postsynaptic neuron classes of interest. Fortunately, this limitation is at least partly surmountable. In cases in which unwanted presynaptic neurons express the photoprobe, it may be possible to identify the presynaptic neuron by the relative position of its cell body and to simulate it selectively using patterned illumination such as that provided by a digital mirror device [18] . In cases in which unwanted postsynaptic neurons are labelled, we have shown that ambiguities can sometimes be resolved using electrophysiological criteria such as the amplitude and time course of membrane current. Restriction of expression patterns using a combinatorial expression system [45] , [46] is another option for addressing this limitation. An alternative method for determining functional connectivity in C. elegans is 'all-optical interrogation', which also employs optogenetic techniques to activate (or inactivate) presynaptic neurons, but uses calcium imaging rather than electrophysiology to monitor postsynaptic neurons [18] . All-optical interrogation is probably better suited for a large-scale, first-pass examination of functional connectivity in which it is advantageous to investigate several pairs of neurons in a single preparation. Other advantages include the ability to resolve activity in subcellular compartments and to preserve both internal milieu and whole-animal behaviour. Photo-electrophysiology is probably better suited for situations in which calcium concentration is an inappropriate proxy for membrane potential or synaptic current. Such situations include separation of the effects of membrane currents from the effects of synaptic currents, as well as the detection and analysis of synaptic inhibition, other subthreshold events, synaptic events that occur on the time scale of milliseconds to tens of milliseconds, and the latency of synaptic transmission. Other advantages include the ability to manipulate cellular and synaptic physiology by altering a neuron's internal or external milieu. The anatomical connectivity of the nervous system of the nematode worm C. elegans has been reconstructed completely [16] , but the signs and strengths of its synaptic connections are almost entirely unknown. Photo-electrophysiology should greatly accelerate the process of annotating the neuronal wiring diagram. Indeed, we used the new approach to characterize the net physiological effects sra-6 -expressing neurons upon the command neuron AVA. The functional connection between these neurons and AVA exhibits three components: an onset transient, a sustained current and an increase in unitary event frequency. We found that all three components are sensitive to glutamate antagonists. In perhaps the simplest interpretation of these findings, the onset transient and the sustained current are the result of temporal summation of the unitary currents, such that all three components are manifestations of a single synaptic mechanism. Under this interpretation, the fact that glutamate blockade is incomplete is explained by incomplete access of the antagonists to the central nervous system, but our experiments do not, of course, exclude the possibility that additional synaptic mechanisms are involved. The conclusion that the functional connection between ASH and AVA is graded is complicated by the possibility that although expression of ChR2 in ASI neurons in XL165 worms is weak, it might be sufficient to generate a significant amount of synaptic current in AVA. If so, it is formally possible that the connection between ASH and AVA is not graded, that is, it is a step function whose effect is balanced by inhibitory effects of the functional connection between ASI and AVA. Although the ASI-AVA connection is likely to be inhibitory as the model requires, we think this scenario is unlikely because the it would require that the effect of ASI-AVA connection to be greatest when ASI is least activated ( Fig. 7 ). 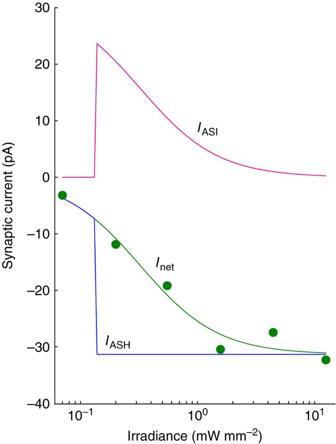Figure 7: Hypothetical current–irradiance curve for the functional connection between ASI and AVA. The model assumes that ASI inhibits AVA (that is, currents attributable to ASI are greater than or equal to zero at all irradiances), which is justified by the fact that ablation of ASI neurons causes an increase in reversal frequency22. The model also assumes, counterfactually, that the current-irradiance curve for the connection between ASH and AVA (blue) is a step function (that is, the connection is not graded).IASI, the predicted curve for the ASI connection (magenta) was computed by subtracting the step functionIASHfromInet(green), the overall current–irradiance curve obtained experimentally. Figure 7: Hypothetical current–irradiance curve for the functional connection between ASI and AVA. The model assumes that ASI inhibits AVA (that is, currents attributable to ASI are greater than or equal to zero at all irradiances), which is justified by the fact that ablation of ASI neurons causes an increase in reversal frequency [22] . The model also assumes, counterfactually, that the current-irradiance curve for the connection between ASH and AVA (blue) is a step function (that is, the connection is not graded). I ASI , the predicted curve for the ASI connection (magenta) was computed by subtracting the step function I ASH from I net (green), the overall current–irradiance curve obtained experimentally. Full size image Graded synaptic transmission between ASH and AVA is consistent with a model in which stronger—and probably more dangerous—aversive stimuli elicit a greater number of stochastic escape responses per unit time. As energetic cost almost certainly increases with the number of escape responses, graded transmission between ASH and AVA may exist to provide a means of reserving the most costly responses for the most dangerous stimuli. Animals The strains used in this study were wild-type C. elegans Bristol (N2), MT7929 unc-13 ( e51 ); CB169 unc-31 ( e169 ); XL157 ntIs29[nmr-1 ∷ tdTomato] , XL153 ntIs27[sra-6 ∷ ChR2*YFP,unc-122 ∷ dsRed] , XL165 ntIs2[sra-6 ∷ ChR2*YFP,unc-122 ∷ dsRED] ; ntIs29[nmr-1 ∷ tdTomato] , XL167 unc-31(e928) ; ntIs27[sra-6 ∷ ChR2*YFP,unc-122 ∷ dsRED] ; ntIs29[nmr-1 ∷ ∷ tdTomato] , XL168 unc-13(e51);ntIs27[sra-6 ∷ ChR2*YFP,unc-122 ∷ dsRED] ; ntIs29[nmr-1 ∷ tdTomato] . NC1749 otEx239[(rig-3 ∷ GFP) , pha-1(e2123)III] ; hdIs32[glr-1 ∷ DsRed2] was a gift from Clay Spencer and David Miller [47] . Molecular biology The sra-6 ∷ ChR2*YFP construct was made by first inserting the sra-6 promoter into the xba-1 site of the pPD95.75 Fire Vector [48] . ChR2*YFP was then inserted between the Bam HI and Eco RI site of pPD95.75 3′ of the promoter. The psra-6 (ref. 8 ) and ChR2*YFP [2] were obtained as clones of preexisting constructs. The nmr-1 ∷ tdTomato plasmid was made by first inserting tdTomato between the Bam HI and Eco R1 sites of pPD95.75. In all, 5 kb of the nmr-1 promoter and the first 5 codons of the predicted nmr-1 protein coding sequence [12] were amplified from genomic DNA by PCR and inserted between the sphI and salI to fuse tdTomato with the first 5 codons of nmr-1 in the pPD95.75 vector. All constructs were injected at 50 ng μl −1 using published methods [48] . Photostimulation Worms were photostimulated in both the behavioural and electrophysiological experiments using the blue channel (470 nm) of a dual-wavelength LED module (Rapp OptoElectronic) that was focused by a 63× 1.4 NA oil immersion objective lens (Zeiss, part number 440762-9904). Irradiance was determined by measuring the power emitted from the objective using an optical power meter placed above the front lens of the objective (Newport) and dividing by the area of the field of illumination at the focal plane of the preparation. Electrophysiology Worms were prepared for electrophysiology by gluing them to an agarose pad formed on a coverslip that became the bottom of the recording chamber as described in ref. 26 . Here, however, the pad contained grooves (cross-section 20 μm×20 μm) formed by pressing a microfabricated polydimethylsiloxane mould [49] into a drop of molten agar to produce an obliquely crossed array ( Fig. 1c ). To ensure that the pad adhered to the coverslip and not to the mould, the coverslip was pre-coated with a thin layer of agarose that was allowed to dry before forming the pad. Prior to gluing, each worm was positioned with its body in one groove and the tip of its head in a second groove that intersected the first one. As a result, the neck region was bent slightly to one side, producing a convex surface at the point of contact between the dissecting probe and the body; this arrangement applies tension to the worm's cuticle to facilitate entry of the sharp glass probe used for dissection. In addition, the worm was rotated so that its ventral midline was at the bottom of the first groove, placing the target neuron at the most favourable latitude for dissection. The chamber was filled with external saline and the cell body of the neuron was exposed by making a small slit in the cuticle. Recording pipettes were pulled and pressure-polished [50] to achieve resistances of 10–20 MΩ when filled with normal internal saline. Voltage- and current-clamp recordings were made with a modified Axopatch 200A [26] amplifier. Pulses used to calculate whole-cell capacitance and series resistance were filtered at 50 kHz and sampled at 125 kHz. Voltage clamp current families, and recordings of photostimulation-evoked events, were filtered at 2 kHz and sampled at 10 kHz. Physiological solutions Internal saline consisted of (in mM): 125 K-gluconate, 1 CaCl 2 , 18 KCl, 4 NaCl, 1 MgCl 2 , 10 HEPES, 10 EGTA, pH 7.2 (KOH). External saline consisted of 5 KCl, 10 HEPES, 8 CaCl 2 , 143 NaCl, 30 glucose, pH 7.2 (NaOH). Behavioural analysis Worms were prepared for behavioural experiments [30] and care was taken to ensure that the conditions of behavioural and electrophysiological experiments were closely matched. Briefly, each worm was glued by the head to an agarose-coated coverslip that formed the bottom of the recording chamber. The preparation was submerged in external physiological saline and positioned on the stage of the inverted microscope normally used for patch clamping and photostimulation; thus, the same microscope objective (×63) and light source were used in both types of experiments. Whole-worm behaviour was recorded (29.97 FPS) using a video camera attached to an ×4 objective stationed above the preparation; the camera was fitted with a long-pass emission filter to prevent the ChR2 excitation light from reaching the camera. Behavioural state (forward or reverse) was scored off-line by noting the direction in which undulatory waves propagated along the worm's body; the scorer was blind to the timing and irradiance of the stimulus as well as the experimental treatment (±all- trans retinal). The time course of the probability of each state was obtained by aligning the behavioural records of different animals to stimulus onset and computing bin-wise averages of the fraction of time spent in each state across animals. Data analysis and statistics Whole-cell capacitance and series resistance were estimated from the currents evoked by a voltage pulse from −40 to −70 mV [26] . Briefly, after seal formation, we measured uncompensated electrode capacitance and seal resistance in the on-cell configuration before rupturing the patch to obtain the whole-cell configuration. The effects of uncompensated electrode capacitance of the current across the seal resistance were removed by subtracting on-cell currents from whole-cell currents before further analysis. The time constant of AVA neurons was estimated as the product of whole-cell capacitance and resistance. Series resistance errors were compensated offline. We excluded cells that had a whole-cell capacitance of less than 0.2 pF, or a holding current at −55 mV that was outside the range of −40 to 20 pA, as these cells were likely to be damaged. In current-clamp experiments, we excluded cells in which the resting potential was less negative than −50 mV. Components of synaptic current The onset transient was quantified as the peak inward current observed during the first 50 ms of the photostimulus minus the peak current observed in the 50 ms immediately before the stimulus. The sustained component of the synaptic current was quantified as the average median-filtered current during the initial 2.1 s of the stimulus minus the average current during an equivalent period immediately before the photostimulus. The frequency of unitary events was defined in terms of events detected, using a weighted least-squares fit of a scaled template. [49] For this component, synaptic response was defined as the frequency of unitary currents during the stimulus, minus the frequency of unitary events during equivalent period immediately before the photostimulus. Analyses were performed using custom software written using IgorPro or the ScyPy [51] Python libraries. Error bars represent±standard error of the mean (s.e.m. ). How to cite this article: Lindsay, T. H. et al . Optogenetic analysis of synaptic transmission in the central nervous system of the nematode C. elegans . Nat. Commun. 2:306 doi: 10.1038/ncomms1304 (2011).